Circadian rhythms in Mexican blind cavefishAstyanax mexicanusin the lab and in the field Biological clocks have evolved as an adaptation to life on a rhythmic planet, synchronising physiological processes to the environmental light–dark cycle. Here we examine circadian clock function in Mexican blind cavefish Astyanax mexicanus and its surface counterpart. In the lab, adult surface fish show robust circadian rhythms in per1 , which are retained in cave populations, but with substantial alterations. These changes may be due to increased levels of light-inducible genes in cavefish, including clock repressor per2 . From a molecular standpoint, cavefish appear as if they experience ‘constant light’ rather than perpetual darkness. Micos River samples show similar per1 oscillations to those in the lab. However, data from Chica Cave shows complete repression of clock function, while expression of several light-responsive genes is raised, including DNA repair genes. We propose that altered expression of light-inducible genes provides a selective advantage to cavefish at the expense of a damped circadian oscillator. Most animals and plants possess endogenous circadian clocks. For these clocks to serve a useful behavioural or physiological purpose, they need to be set or entrained to local time, and the most common resetting signal, or zeitgeber, is the environmental light–dark (LD) cycle. Indeed, circadian clocks are fundamentally an adaptation to life on a rhythmic planet. It has therefore been the generally held view that cave or deep sea animals that have evolved in a constant dark environment have no need for a functional clock and, in fact, no longer possess one. Although this makes apparent sense, there are relatively few studies that have examined circadian clocks in cave species, less that have studied the molecular nature of these clocks and none that have done so under native cave conditions in the wild [1] , [2] , [3] , [4] , [5] , [6] , [7] , [8] , [9] . The blind Mexican cavefish, Astyanax mexicanus , is an important model system for the study of numerous adaptive and regressive evolutionary changes that have occurred as animals have evolved to life underground. These changes include the loss of functional eyes and pigmentation, two regressive traits that are common to most cave species [10] , [11] , [12] , [13] . Astyanax has several major advantages for such studies, not least the fact that direct descendants of ancestral surface fish persist within the neighbouring rivers of the Sierra de El Abra region of North East Mexico [14] , [15] . This makes it possible to determine how a given biological process has evolved in constant darkness, even down to specific molecular changes, by comparing directly descendants of the founding river fish with isolated cave populations. In addition, there are numerous distinct and well-defined cave strains of Astyanax in this region of Mexico, making it possible to compare the evolution of specific traits amongst several independent populations [14] , [15] , [16] , [17] . As such, Astyanax mexicanus provides a unique opportunity to explore how the circadian clock has changed between river and cave following several hundred thousand years or more of constant darkness. Much of what is known about teleost molecular clocks comes from studies in zebrafish. Independent circadian clocks are found in virtually all zebrafish tissues, and these tissues are themselves directly light responsive [18] , [19] . Light signals have a strong impact, not only on resetting of the zebrafish circadian clock [20] , [21] , [22] , but also on numerous aspects of zebrafish cell biology, such as the activation of DNA repair processes [23] , [24] , [25] , [26] and the regulation of cell cycle events [27] , [28] , [29] , [30] . Evolving in a completely dark environment is therefore likely to impact fish physiology in a dramatic manner. The highly decentralized nature of teleost clocks is an important aspect of our studies on Astyanax circadian rhythms, as it has allowed us to explore clock function using fin clips taken from animals at different circadian times, in the laboratory and in the field. This fact has proved essential due, in part, to the scarcity of these animals and the difficulty in obtaining samples, especially under natural conditions in the wild. The results of this study show a robust circadian oscillation in period1 (per1) gene expression in surface fish in the lab, as well as in the field; this oscillation is also present in two cave populations of Astyanax following light entrainment in the lab, but with considerable differences in the waveform of the rhythm. In addition, the light input pathway is clearly altered following evolution in the cave with the expression of several light-inducible genes, including the clock repressor per2 and DNA repair genes, present at raised basal levels in cavefish; this is particularly true for individuals sampled under natural conditions within the cave itself, where no molecular clock gene rhythms are detected. These results support the idea that cavefish do not use a clock underground, but instead, possess tonically activated light-dependent processes, including enhanced DNA repair. 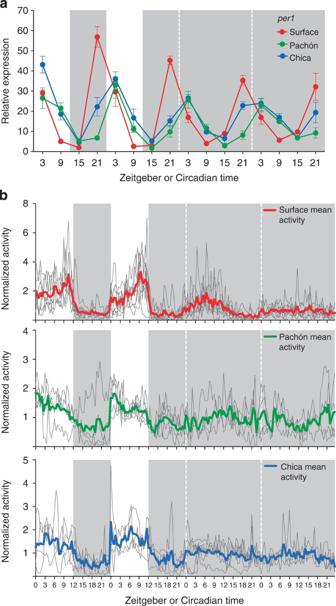Figure 1: Molecular and behavioural analysis of cavefish reveals an altered circadian oscillator. (a) Adult fish were entrained to a LD cycle for 7 days and transferred into constant darkness. Fin samples were taken every 6 h at the indicated zeitgeber or circadian times (ZT or CT), where ZT0 is lights on.Per1mRNA levels were measured by qPCR and normalized to the reference generpl13α. Relative expression was calculated and plotted using the ΔΔCtmethod. Rhythm amplitude was estimated by averaging peak to trough values in LD, and was 20.61-fold for surface, 7.71-fold for Pachón and 8.26-fold for Chica. White and grey shaded areas indicate light and dark periods, respectively. Data represent the mean±s.e.m. of at least four different fish. (b) Adult fish were kept in individual tanks with an IR camera mounted above. Fish were entrained to a LD cycle for 7 days and transferred into constant darkness for 2 days. Filming took place over the final 2 days in LD and first 2 days in constant darkness. The time spent in seconds swimming at a velocity of greater than 5 cm s−1per 30 min bin was extracted from each video file. Data were normalized for each fish filmed. Data plotted represent the average, as well as individual traces, of normalized activity for four or more fish. All three populations show significant 24 h rhythms in LD as determined by autocorrelation, and estimates of period (shown in the text) were determined by spectrum resampling38. Rhythms of locomotor activity are present in constant darkness in surface fish, but are not present in either cavefish. Isolation of circadian clock genes from Astyanax mexicanus To determine whether cavefish have a functional circadian clock, we isolated several clock genes from surface, Pachón and Chica strains of Astyanax , including full-length coding sequences for per1 and cryptochrome 1a ( cry1a ), as well as a partial sequence for per2 ( Table 1 and Supplementary Fig. S1 ). Per1 represents a key element of the core clock mechanism and, in most teleosts studied to date, shows high-amplitude circadian oscillations [20] , [31] , [32] . Per1 is therefore an excellent marker of clock function. Cry1a and per2 have been shown in teleosts to be important for light resetting of the circadian clock [22] , [33] . These genes are primarily regulated by light and are thus good markers of light sensitivity [22] , [34] , [35] , [36] . Sequence analysis reveals a high degree of conservation between the three populations of Astyanax in all clock genes isolated. This greatly simplified our molecular analysis (described below) and permitted the use of one set of gene-specific primers, instead of three (one for each fish population), for quantitative polymerase chain reaction (qPCR). Table 1 Comparison of A. mexicanus gene sequences. Full size table Comparison of the predicted clock protein sequences showed a remarkable degree of similarity. For example, of the thirteen amino-acid changes in Pachón PER1 compared with the surface fish protein, twelve of these changes are identical between the two cave strains, Pachón and Chica. A similar comparison of the light-inducible CRY1a protein reveals 5 amino-acid differences, all of which are identical in the two cave populations ( Supplementary Fig. S1 ). This level of sequence similarity between different cave populations seems unusual, as it has been proposed that animals from the El Abra cluster of caves have arisen from independent invasions of the underground environment, though this is a topic of some debate [12] , [14] , [37] . The differences between cave and surface fish sequences, however, may simply represent more recent changes to the surface genome from the original river ancestor, rather than cave-specific evolutionary changes. Rhythmic expression of per1 in cavefish in the lab To determine whether Astyanax cave populations still retain a functional circadian clock, adult surface fish, Pachón and Chica cavefish were entrained to a 12/12-hour LD cycle under laboratory conditions, and fins were clipped at 6-hour intervals. After 2 days of collecting samples on a LD cycle, the animals were allowed to ‘free-run’ into constant darkness (DD), with sampling continuing for a further two cycles. Samples were analysed by qPCR to determine the levels of per1 messenger RNA (mRNA). Figure 1a shows that caudal fin samples from surface fish have a high-amplitude rhythm in per1 expression, with a peak in the late night at zeitgeber time (ZT) 21. This rhythm continues robustly as the animals free-run into DD ( Fig. 1a and Supplementary Fig. S2 ). Per1 levels also oscillate in the two cave populations, showing that cavefish retain the ability to detect light and generate molecular circadian oscillations. However, there are clear and consistent differences between the rhythms seen in surface and cave populations. First, the cavefish per1 rhythm is lower in amplitude, with a relative peak to trough ratio in LD of 7.71- and 8.26-fold in Pachón and Chica, respectively, compared with 20.61-fold in surface fish. Secondly, the timing or entrained phase of the per1 rhythm is clearly different, with peak expression occurring 6 h later in both cave populations. These differences then persist in DD ( Fig. 1a and Supplementary Fig. S2 ). Figure 1: Molecular and behavioural analysis of cavefish reveals an altered circadian oscillator. ( a ) Adult fish were entrained to a LD cycle for 7 days and transferred into constant darkness. Fin samples were taken every 6 h at the indicated zeitgeber or circadian times (ZT or CT), where ZT0 is lights on. Per1 mRNA levels were measured by qPCR and normalized to the reference gene rpl13 α. Relative expression was calculated and plotted using the ΔΔ C t method. Rhythm amplitude was estimated by averaging peak to trough values in LD, and was 20.61-fold for surface, 7.71-fold for Pachón and 8.26-fold for Chica. White and grey shaded areas indicate light and dark periods, respectively. Data represent the mean±s.e.m. of at least four different fish. ( b ) Adult fish were kept in individual tanks with an IR camera mounted above. Fish were entrained to a LD cycle for 7 days and transferred into constant darkness for 2 days. Filming took place over the final 2 days in LD and first 2 days in constant darkness. The time spent in seconds swimming at a velocity of greater than 5 cm s −1 per 30 min bin was extracted from each video file. Data were normalized for each fish filmed. Data plotted represent the average, as well as individual traces, of normalized activity for four or more fish. All three populations show significant 24 h rhythms in LD as determined by autocorrelation, and estimates of period (shown in the text) were determined by spectrum resampling [38] . Rhythms of locomotor activity are present in constant darkness in surface fish, but are not present in either cavefish. Full size image To determine whether these molecular rhythms are reflected in an output of the circadian clock, we monitored the swimming behaviour of surface and two cave populations. Adult fish were entrained to a LD cycle as above and then transferred into DD, and locomotor activity was recorded over a 4-day period (2 days of LD into 2 days of DD). Analysis of burst activity (velocity >5 cm s −1 ) reveals significantly weaker circadian rhythms in cavefish compared with surface fish, as determined by autocorrelation and spectrum resampling [38] . These results are consistent with the molecular alterations in per1 expression and the somewhat less robust clock function observed above ( Fig. 1 ). Surface fish show a clear, diurnal circadian rhythm in swimming behaviour in LD (23.95±1.01 h), which persists on the first day in DD (29.77±2.49 h), but then essentially becomes arrhythmic on the second day in DD ( Fig. 1b ). Pachón and Chica cavefish also show significant circadian rhythms in LD (23.95±0.82 h and 25.6±1.30 h, respectively), but after entry into DD, both populations are behaviourally arrhythmic and show substantial variation between individuals. Interestingly, cavefish activity remains at median to peak levels in DD, whereas surface fish activity drops closer to basal lower levels ( Fig. 1b ). These results are consistent with previous behavioural studies of Astyanax , which showed that cavefish had higher activity in the night and therefore appeared to sleep less than surface fish [1] , [3] , [5] . Together, these molecular and behavioural data reveal that cavefish do possess a functional circadian clock, but one that is distinctly less robust than that of the surface river population. Alteration in light induction of per2 repressor in cavefish The differences we observe in rhythm amplitude and phase angle of per1 expression between surface and cave strains could be a consequence of changes within the core clock mechanism that generates the oscillation, alterations in the light input pathway or, of course, both. From work in zebrafish, several light-induced genes, including cry1a and per2 , are known to be critical for light resetting of the circadian pacemaker [22] , [33] . Astyanax cave strains are able to entrain to some extent to laboratory LD conditions, as we have shown above, but impairment of the input pathway could lead to a less robust rhythm through weaker cell synchronization, as well as changes in the phase angle between the clock and the LD cycle. So is the light input pathway altered in cave populations of Astyanax ? To address this question, we examined the induction of both cry1a and per2 mRNA in Astyanax mexicanus , following a 3-hour light pulse applied to whole fish in the early evening at ZT16 ( Fig. 2a,c ). The expression of cry1a and per2 is strongly induced in surface fish, similar to previous reports in zebrafish [22] , [34] , [35] , [36] . This acute light response is greatly reduced, though still statistically significant, in Pachón cavefish and does not occur in Chica cavefish. Interestingly, rather than a change in the actual light-induced levels, this reduction or absence of a light response is due to significantly raised basal expression in the dark control samples of cavefish compared with surface individuals. In cavefish, cry1a and per2 are present at near maximal levels in the absence of any light stimulus. 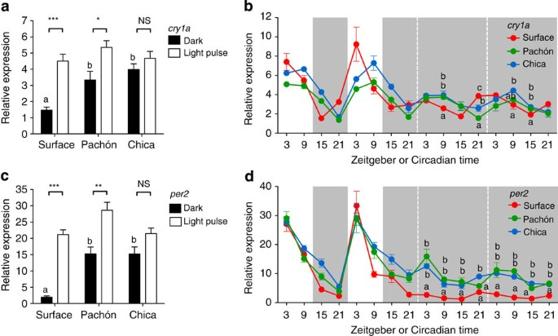Figure 2: Acute induction of light-inducible genes is reduced in cavefish due to increased basal expression levels. Adult fish were entrained on a LD cycle for 7 days and given a 3 h light pulse at ZT16. Expression ofcry1a(a) andper2(c) was determined in light-pulsed and dark control fin samples by qPCR and normalized to the reference generpl13α. Relative expression levels were calculated and plotted using the ΔΔCtmethod. Dark- and light-induced levels ofcry1aandper2were compared using a Student’st-test (unpaired, two tailed; *P<0.05; **P<0.01; ***P<0.001). Dark levels ofcry1aandper2were compared between all populations using ANOVA followed by Newman–Keuls multiple comparison tests. Different lower case letters indicates significant differences between comparisons.Cry1a(b) andper2(d) mRNA levels were determined by qPCR in the same samples asFig. 1. White and grey shaded areas indicate light and dark periods, respectively. Expression levels ofcry1aandper2were compared between all populations at each time point in DD by ANOVA followed by Newman–Keuls multiple comparison tests. Different lower case letters indicate significant differences between comparisons. Data represent the mean±s.e.m. from at least four different fish. Figure 2: Acute induction of light-inducible genes is reduced in cavefish due to increased basal expression levels. Adult fish were entrained on a LD cycle for 7 days and given a 3 h light pulse at ZT16. Expression of cry1a ( a ) and per2 ( c ) was determined in light-pulsed and dark control fin samples by qPCR and normalized to the reference gene rpl13 α. Relative expression levels were calculated and plotted using the ΔΔ C t method. Dark- and light-induced levels of cry1a and per2 were compared using a Student’s t -test (unpaired, two tailed; * P <0.05; ** P <0.01; *** P <0.001). Dark levels of cry1a and per2 were compared between all populations using ANOVA followed by Newman–Keuls multiple comparison tests. Different lower case letters indicates significant differences between comparisons. Cry1a ( b ) and per2 ( d ) mRNA levels were determined by qPCR in the same samples as Fig. 1 . White and grey shaded areas indicate light and dark periods, respectively. Expression levels of cry1a and per2 were compared between all populations at each time point in DD by ANOVA followed by Newman–Keuls multiple comparison tests. Different lower case letters indicate significant differences between comparisons. Data represent the mean±s.e.m. from at least four different fish. Full size image We then examined in more detail cry1a and per2 expression in DD, following entrainment to a LD cycle. The results show that rhythmic expression of cry1a persists in DD, but that for most time points, these levels are not significantly different between surface and cavefish ( Fig. 2b ). In contrast, per2 expression is primarily light-regulated and, at best, weakly clock-controlled, as reported for zebrafish [34] , [36] ( Fig. 2d ). More interestingly, however, is the fact that per2 is present at significantly raised levels in cave strains compared with surface fish in DD. As per2 is a light-induced clock repressor and is thought to be important for clock entrainment in fish systems [33] , [36] , this level of increased tonic expression could explain, at least in part, the reduced amplitude and altered phase of molecular clock rhythms in cave populations. We know that overexpression of per2 in zebrafish cell lines has a significant damping effect on per1 rhythms ( Supplementary Fig. S3 ), which is also true for overexpression of cry1a [22] . Thus, there is a clear perturbation of the light input pathway in cave populations of Astyanax mexicanus , with the light-responsive per2 gene constitutively expressed at high levels. We next examined the expression of thyrotroph embryonic factor 1 ( tef1 ), which lies upstream of per2 and is itself a light-inducible gene in zebrafish [25] , [26] . TEF1 is a transcriptional activator and belongs to the family of bZIP PAR domain containing DNA binding proteins, which recognize D-box regulatory sequences (TTAYGTAA or TTATACAA). Zebrafish TEF1 has been shown to bind directly to a D-box element in the per2 promoter and transcriptionally activate its expression in response to light [36] , [39] . We therefore cloned tef1 from surface and cave populations of Astyanax to determine whether it might contribute to the upregulation of per2 in cavefish. Our results, however, show no significant light induction for tef1 at ZT16 in any population of Astyanax , including surface fish ( Supplementary Fig. S4a ). A relatively weak light induction is detected at CT0 in surface and Pachón fish, but not in Chica cavefish ( Supplementary Fig. S4b ). Moreover, the basal levels of tef1 expression are not significantly raised above those in surface fish, with the possible exception in Chica at CT0. Together these results do not support the hypothesis that raised upstream levels of tef1 expression are responsible for the constitutively high levels of per2 in cavefish. However, we cannot exclude the possibility that the TEF1 protein, rather than its mRNA, or another D-box binding factor is contributing to the light signalling pathway. In the Somalian cavefish, Phreatichthys andruzzii , proteins implicated in circadian light detection, in particular teleost multiple tissue (TMT) opsin and melanopsin, appear to have carboxy-terminal truncations that would impair their role as functional photopigments. An examination of the tmt opsin sequence between surface and Pachón shows no such truncations in Astyanax ( Supplementary Fig. S5a ). Furthermore, the levels of tmt opsin expression appear similar between surface and Chica cavefish, with a slight reduction in Pachón ( Supplementary Fig. S5b ). Therefore, this upstream aspect of the light sensing biology of Astyanax does not appear to be significantly altered. Changes in cavefish clock partially reversed in hybrid fish Astyanax surface and cave strains belong to the same species and, as such, may be crossed within different populations to produce F1 hybrid offspring. We therefore generated F1 surface x Pachón hybrid fish and explored further the circadian light input pathway in adult hybrid animals. Light induction of both cry1a and per2 in response to a 3-hour light pulse is virtually restored in the hybrid fish, though the absolute levels of cry1a mRNA are slightly reduced in hybrids ( Fig. 3a,b ). Cry1a is induced 3.07-fold in surface fish compared with 2.72-fold in the hybrid and 1.60-fold in Pachón, whereas per2 is induced 10.91-fold in surface, 10.36-fold in the hybrid and 1.88-fold in Pachón. Interestingly, the raised basal levels of cry1a and per2 found in Pachón fish are completely suppressed to surface fish levels in the F1 hybrids ( Fig. 3a,b ). 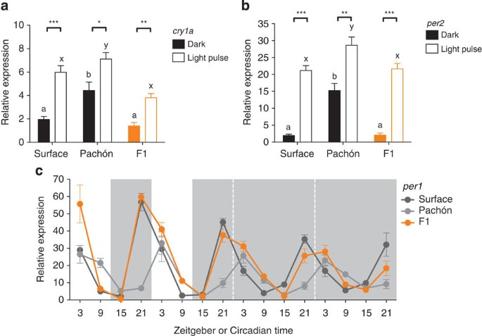Figure 3: The acute light response and circadian entrainment are restored in F1 hybrid fish. Adult F1 surface x Pachón hybrid fish were entrained to a LD cycle and given a 3 h light pulse at ZT16. Expression levels ofcry1a(a) andper2(b) were determined in light-pulsed and dark control fin samples by qPCR (orange), and compared with both surface fish and Pachón cavefish (reproduced in grey fromFig. 3). Dark- and light-induced levels ofcry1aandper2were compared using a Student’st-test (unpaired, two tailed; *P<0.05; **P<0.01; ***P<0.001). Dark and light levels ofcry1aandper2were compared between all fish using ANOVA followed by Newman–Keuls multiple comparison tests. Different lower case letters indicates significant differences between comparisons. (c)Per1mRNA levels in F1 hybrid fish were determined by qPCR (orange) and compared with both surface fish and Pachón cavefish (reproduced in grey fromFig. 2).Per1amplitude was estimated by averaging peak to trough ratios in LD, and was 20.61-fold for surface, 35.24-fold for F1 hybrid and 7.71-fold for Pachón. White and grey shaded areas indicate light and dark periods, respectively. Data represent the mean±s.e.m. of at least four different fish. Figure 3: The acute light response and circadian entrainment are restored in F1 hybrid fish. Adult F1 surface x Pachón hybrid fish were entrained to a LD cycle and given a 3 h light pulse at ZT16. Expression levels of cry1a ( a ) and per2 ( b ) were determined in light-pulsed and dark control fin samples by qPCR (orange), and compared with both surface fish and Pachón cavefish (reproduced in grey from Fig. 3 ). Dark- and light-induced levels of cry1a and per2 were compared using a Student’s t -test (unpaired, two tailed; * P <0.05; ** P <0.01; *** P <0.001). Dark and light levels of cry1a and per2 were compared between all fish using ANOVA followed by Newman–Keuls multiple comparison tests. Different lower case letters indicates significant differences between comparisons. ( c ) Per1 mRNA levels in F1 hybrid fish were determined by qPCR (orange) and compared with both surface fish and Pachón cavefish (reproduced in grey from Fig. 2 ). Per1 amplitude was estimated by averaging peak to trough ratios in LD, and was 20.61-fold for surface, 35.24-fold for F1 hybrid and 7.71-fold for Pachón. White and grey shaded areas indicate light and dark periods, respectively. Data represent the mean±s.e.m. of at least four different fish. Full size image An examination of per1 rhythmicity in the hybrid population shows that both the amplitude and entrained phase of the oscillation now match the surface fish population ( Fig. 3c ). The reduced amplitude, as well as the 6-hour delay in per1 timing, observed in the Pachón strain have both been reversed within one generation. When these hybrid animals are allowed to free-run into DD for 2 days, both the amplitude and phase are intermediate between surface and Pachón per1 oscillations ( Fig. 3c ), though more cycles at higher resolution would be needed to make conclusive statements about oscillator period. These results indicate that alterations in the entrainment pathway are recessive and reversed within one cross or generation. However, changes in core oscillator function appear to be more complex and reside at some intermediate state in hybrid animals. This may simply reflect the greater complexity of the clock mechanism and consequently, the greater potential for molecular alterations. Expression of per1 is strongly repressed in wild cavefish Studying cavefish circadian biology in the laboratory, especially following light entrainment, is obviously an unnatural scenario and does not address the more relevant question of what is happening in the caves themselves. We have therefore attempted, over several seasons of field trips to Mexico, to follow circadian clock function under natural conditions in the river and cave. Surface fish were fin-clipped in the Micos River (+22° 6′ 59.01′ N, -99° 10′ 16.8′ W) at six time points per day over 2 days. 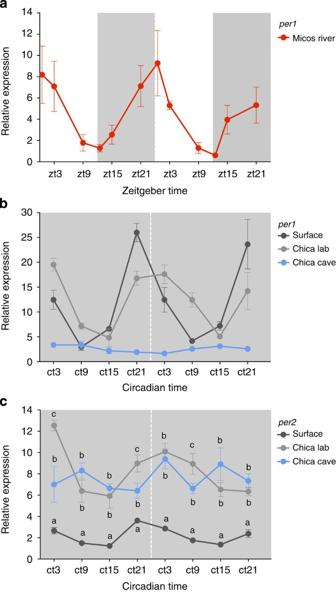Figure 4: Circadian clock gene expression is dramatically altered in cavefish in the wild. (a) Fin samples from surface fish from the Micos River were collected at six time points per day over 2 days.Per1expression levels were measured by qPCR and normalized torpl13α. Relative expression levels were calculated and plotted using the ΔΔCtmethod. White and grey shaded areas indicate light and dark periods, respectively. (b) Chica fin samples were collected in the wild every 6 h over 2 days.Per1mRNA levels are shown in blue and plotted relative to constant dark samples from surface and Chica cavefish entrained in the laboratory for comparison (reproduced in grey fromFig. 1a). (c) Chica fin samples were collected in the wild every 6 h over 2 days.Per2expression levels were measured by qPCR and normalized to the reference generpl13α. Data shown in blue are plotted relative to constant dark samples from laboratory-entrained surface and Chica cavefish for comparison (reproduced in grey fromFig. 2). Expression levels were compared between all populations at each time point in DD by ANOVA followed by Newman–Keuls multiple comparison tests. Different lower case letters indicate significant differences (P<0.05) between comparisons.Per2is significantly more expressed in Chica samples from both the lab and field compared with surface fish. Data represent the mean±s.e.m. from at least four different fish. Figure 4a shows the rhythm in per1 expression in this wild population of Astyanax mexicanus . The relative timing of the oscillation matches that seen under laboratory conditions, with per1 peaking roughly in the late night/early morning and reaching a low point of expression in the early evening, just after sunset. Figure 4: Circadian clock gene expression is dramatically altered in cavefish in the wild. ( a ) Fin samples from surface fish from the Micos River were collected at six time points per day over 2 days. Per1 expression levels were measured by qPCR and normalized to rpl13 α. Relative expression levels were calculated and plotted using the ΔΔ C t method. White and grey shaded areas indicate light and dark periods, respectively. ( b ) Chica fin samples were collected in the wild every 6 h over 2 days. Per1 mRNA levels are shown in blue and plotted relative to constant dark samples from surface and Chica cavefish entrained in the laboratory for comparison (reproduced in grey from Fig. 1a ). ( c ) Chica fin samples were collected in the wild every 6 h over 2 days. Per2 expression levels were measured by qPCR and normalized to the reference gene rpl13 α. Data shown in blue are plotted relative to constant dark samples from laboratory-entrained surface and Chica cavefish for comparison (reproduced in grey from Fig. 2 ). Expression levels were compared between all populations at each time point in DD by ANOVA followed by Newman–Keuls multiple comparison tests. Different lower case letters indicate significant differences ( P <0.05) between comparisons. Per2 is significantly more expressed in Chica samples from both the lab and field compared with surface fish. Data represent the mean±s.e.m. from at least four different fish. Full size image The majority of our cave studies have focused to date on the Chica Cave, 10 km south of Ciudad Valles in the Mexican state of San Luis Potosí (+21° 51′ 36.05’ N, -98° 56′ 10.00’ W). Of all the caves examined, we believe that this location has the highest probability of containing a rhythmic population of fish, mainly due to the large, clearly rhythmic bat population ( Supplementary Fig. S6 ). However, as can be seen in Fig. 4b , for samples collected every 6 h over 2 days, there is no significant oscillation in the levels of per1 expression. After several years of sampling in this location, the combined data support the conclusion that Astyanax in this cave does not show an entrained molecular oscillation. In addition, the expression levels of per1 are significantly lower in cave animals under natural conditions than those measured in surface fish, or equivalent cave strains within the lab. In contrast, the expression of per2 in the cave field samples is significantly raised, similar to the levels observed for cavefish in the lab ( Fig. 4c ). We believe that this lack of rhythmicity is unlikely to be due to the absence of sufficiently strong entraining signals within the cave, since in a rhythmic, but asynchronous population of individuals, one would predict per1 expression to be close to an intermediate level, which we do not observe. Rather, the core clock mechanism is tonically repressed or damped in the cave, probably as a consequence of overactivation of the light input pathway. DNA repair gene expression is altered in cavefish One of the most significant molecular changes between surface and cave populations of Astyanax appears to be light signalling to the circadian clock, and in particular, the raised basal levels of per2 . Could there be some selective advantage of tonically activating the light input pathway? To explore this question, we examined another biological process, DNA repair, previously shown to be light-dependent in teleosts. Several genes encoding DNA repair proteins have been shown in zebrafish to be transcriptionally activated by light [23] , [25] , [26] . Without this light-dependent induction, animals appear to have reduced tolerance to environmental stress and increased mortality [23] , [40] . We isolated two DNA repair genes from populations of Astyanax mexicanus : CPD photolyase (CPD phr) , involved in photoreactivation, and damage-specific DNA binding protein 2 (ddb2) , part of the nucleotide excision repair pathway. Consistent with previous studies in zebrafish [25] , [26] , CPD phr is strongly induced after a 3-hour light pulse in surface fish ( Fig. 5a ). Similar to cry1a and per2 ( Fig. 2 ), CPD phr is also induced by light in cavefish, but with a lower magnitude, because of significantly raised basal expression in dark control samples. An analysis of rhythmic expression of CPD phr after entrainment to a LD cycle reveals raised levels in Pachón and Chica cavefish in constant darkness ( Fig. 5b ). Similar results are seen for ddb2 , particularly in Chica cavefish, where expression is significantly higher than surface fish at seven of the eight time points in constant darkness ( Fig. 5c ). This enhancement of DNA repair gene expression is even more exaggerated within the cave itself ( Fig. 5d,e ). Expression of both CPD phr and ddb2 is dramatically increased in wild cavefish compared with either surface fish, or even cavefish within the laboratory ( Fig. 5d,e ). 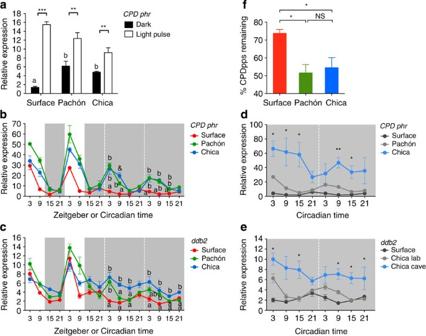Figure 5: Cavefish show enhanced DNA repair gene expression and activity in the dark. (a) Adult fish were entrained to a LD cycle and given a 3-hour light pulse at ZT16.CPD photolyaseexpression levels were determined in light-pulsed and dark control fin samples by qPCR. Dark and light-induced levels ofCPD photolyasewere compared using a Student’st-test (unpaired, two tailed; **P<0.01; ***P<0.001). Dark levels ofCPD photolyasewere compared between all populations using ANOVA followed by Newman–Keuls multiple comparison tests. Different lower case letters indicate significant differences between comparisons. (b,c) Adult fin samples were the same as inFigure 1a.CPD photolyase(b) andddb2(c) mRNA levels were determined by qPCR. White and grey shaded areas indicate light and dark periods, respectively. Data represent the mean±s.e.m. from at least four different fish. Expression ofCPD photolyaseandddb2was compared between all populations after transfer into constant darkness using ANOVA followed by Newman–Keuls multiple comparison tests. Different lower case letters indicates significant differences between comparisons. (d,e) Chica fin samples were collected in the wild every 6 h for 2 days. Expression ofCPD photolyase(d) andddb2(e) are shown in blue and plotted relative to constant dark samples from laboratory-entrained surface and Chica cavefish for comparison (reproduced in grey fromFig. 5b,c). Expression levels ofCPD photolyaseandddb2were compared between surface and wild Chica cavefish at each time point by using a Student’st-test (unpaired, two tailed; *P<0.05; **P<0.01; ***P<0.001). (f) CPD photoproducts (CPDpp) remaining in DNA extracted from adult fins 24 h after a UV light pulse (1 mJ cm−2, 2 s) as calculated by ELISA. Data are shown as a percentage of CPDpp at 24 h with respect to CPDpp present in DNA extracted 0.5 h after the UV pulse. The percentage of CPDpp remaining at 24 h was compared between all populations by ANOVA followed by Newman–Keuls multiple comparison tests. Data represent the mean±s.e.m. from four different fish. Figure 5: Cavefish show enhanced DNA repair gene expression and activity in the dark. ( a ) Adult fish were entrained to a LD cycle and given a 3-hour light pulse at ZT16. CPD photolyase expression levels were determined in light-pulsed and dark control fin samples by qPCR. Dark and light-induced levels of CPD photolyase were compared using a Student’s t -test (unpaired, two tailed; ** P <0.01; *** P <0.001). Dark levels of CPD photolyase were compared between all populations using ANOVA followed by Newman–Keuls multiple comparison tests. Different lower case letters indicate significant differences between comparisons. ( b , c ) Adult fin samples were the same as in Figure 1a . CPD photolyase ( b ) and ddb2 ( c ) mRNA levels were determined by qPCR. White and grey shaded areas indicate light and dark periods, respectively. Data represent the mean±s.e.m. from at least four different fish. Expression of CPD photolyase and ddb2 was compared between all populations after transfer into constant darkness using ANOVA followed by Newman–Keuls multiple comparison tests. Different lower case letters indicates significant differences between comparisons. ( d , e ) Chica fin samples were collected in the wild every 6 h for 2 days. Expression of CPD photolyase ( d ) and ddb2 ( e ) are shown in blue and plotted relative to constant dark samples from laboratory-entrained surface and Chica cavefish for comparison (reproduced in grey from Fig. 5b,c ). Expression levels of CPD photolyase and ddb2 were compared between surface and wild Chica cavefish at each time point by using a Student’s t -test (unpaired, two tailed; * P <0.05; ** P <0.01; *** P <0.001). ( f ) CPD photoproducts (CPDpp) remaining in DNA extracted from adult fins 24 h after a UV light pulse (1 mJ cm −2 , 2 s) as calculated by ELISA. Data are shown as a percentage of CPDpp at 24 h with respect to CPDpp present in DNA extracted 0.5 h after the UV pulse. The percentage of CPDpp remaining at 24 h was compared between all populations by ANOVA followed by Newman–Keuls multiple comparison tests. Data represent the mean±s.e.m. from four different fish. Full size image To examine whether this increase in gene expression confers greater DNA repair activity in the dark, we measured DNA damage after UV exposure. Adult surface fish and cavefish were maintained on a LD cycle. Fin clips were then collected at ZT23, placed into culture and exposed to 1 mJ cm −2 of UV light for 2 s. Samples were then incubated in the dark for 24 h, and genomic DNA was extracted from UV-treated fins and untreated controls. To assess DNA damage, we performed an enzyme-linked immunosorbent assay (ELISA) using an antibody to CPD photoproducts [41] . The results show significantly lower DNA damage, and therefore higher DNA repair activity, in Pachón and Chica cavefish compared with surface fish even in the dark ( Fig. 5f ). Importantly, this demonstrates that the raised levels of DNA repair gene expression in cavefish results in an improved ability to repair UV-damaged DNA. Furthermore, as gene expression levels are higher in wild cavefish, it suggests that DNA repair activity would be even greater in the caves. Astyanax mexicanus has established itself as an important evolutionary model system for the study of a wide variety of biological processes, not least because direct descendants of the ancestral surface dwelling form coexist with multiple isolated cave forms [14] , [15] . This allows direct molecular and physiological comparisons to be made between surface and cave individuals of the same species, and statements to be made about how these processes have changed after hundreds of thousands of years in complete darkness. In this study, we have explored, under both laboratory and field conditions, how the circadian clock has evolved in this species. In the laboratory, surface fish show a robust circadian oscillation in per1 gene expression, as has been previously reported for zebrafish and other teleost species [20] , [31] , [32] , [34] , [42] . A high-amplitude per1 rhythm is also apparent in surface fish under natural conditions. These samples were collected in the Micos River in March, when the sunrise and sunset times create an almost perfect 12/12-hour LD cycle, with temperature fluctuations in the river no greater than 0.5 °C. The fundamental timing of the oscillation is very similar to that observed in the lab, but not surprisingly, there is greater variation within the wild animal data set. There are several possible explanations for this, including greater genetic variation in the wild compared with the lab population, as well as differences in animal health and age, light intensity and spectral quality at the water surface of Micos River ( Supplementary Fig. S7 ). Together, these factors will impact gene expression patterns under natural conditions. Interestingly, cavefish have the capacity to generate molecular oscillations in the lab, but no per1 rhythms were detected over a 2-day sampling period in Chica Cave. These data are representative of results collected over several years of fieldwork in this particular cave, between 2007 and 2010. In our opinion, the environment within Chica Cave is the most likely to be rhythmic and to possess daily timing cues in the wild due to a large and highly rhythmic bat population, which displays clear bursts of activity around dawn and dusk as they enter and leave the cave ( Supplementary Fig. S6 ). The bats spiral over the underground ponds prior to exiting, and we hypothesized that this activity may provide an entraining signal to the fish in a variety of ways, including providing a feeding cue through rhythmic defecation. However, our per1 expression analysis has failed to produce any evidence that this occurs. Therefore, rhythmic bat activity and a likely feeding cue they might provide do not appear to be a sufficient zeitgeber to entrain the circadian clock under natural conditions. In our opinion, a lack of overt clock function at this location makes it highly unlikely that other cave populations, such as Pachón, where there are even fewer possible entraining signals, will show any circadian rhythmicity. In the laboratory, consistent differences in per1 expression exist between surface and cave populations, the most striking of which is a clear delay in the phase of the per1 rhythm relative to the LD cycle in cave animals. The amplitude of the rhythm also appears reduced. Per1 expression in the cave field samples is, in fact, much lower than that seen in surface fish or in cave strains in the lab ( Fig. 4b ). This very low transcript level is unlikely to be the consequence of simple asynchrony or lack of clock entrainment, but more reasonably reflects actual repression of core clock function. These results support the hypothesis that the oscillator is actually not ‘running’ under these conditions. Constant light has been shown in zebrafish to ‘stop’ the circadian oscillator and overexpression of both cry1a and per2 genes mimic this action of light [22] . The CRY1a and PER2 proteins act as strong repressors of CLOCK-BMAL transcriptional activity, leading to a decrease in per1 gene expression, and ‘stopping’ the clock when overexpressed or induced by sustained light exposure. Both of these genes appear to be important for clock entrainment [22] , [33] . The basally increased levels, particularly of per2 in cavefish, are likely to do the same, leading to the extremely reduced per1 expression we detect under natural conditions. It is highly likely that these molecular changes in the light input pathway also contribute to the phase differences observed between surface and cave populations in the lab, and especially to the reduced amplitude of the core clock oscillation. These results lead us to conclude that the light input pathway exists in a more activated state in cave populations, as if the fish were actually experiencing constant light rather than the perpetual darkness of the cave. Clock-controlled locomotor rhythms are absent in cavefish in DD, following entrainment on a LD cycle. This corroborates previous work on locomotor rhythms in Astyanax , which suggests a significant reduction or lack of rhythmic behaviour in cavefish [3] , [5] . Cavefish activity in LD is weakly rhythmic, with a general increase in the day, which probably represents a masking influence of the light on their behaviour. These data raise the interesting possibility that in cavefish, the molecular circadian rhythm is somehow uncoupled from the control of locomotor activity and possibly other outputs of the clock. An analysis of additional clock-regulated outputs in this system will be required to confirm whether this phenomenon is specific to just locomotor behaviour or extends more widely to other clock-controlled processes. In addition, such a conclusion would benefit from a considerably greater understanding of how the core clock mechanism actually links to the regulation of different outputs in fish. It is interesting to note that previous studies on cave animals, such as amphipods and salamanders, have examined behaviour to suggest that circadian rhythms are lost [9] , [43] . It would be interesting to re-examine those species at the molecular clock level in the light of the gene expression data presented here. The circadian phenotypes we observe in Astyanax cavefish are much less drastic than those recently reported for the Somalian cavefish, Phreatichthys andruzzii , which have completely lost the ability to entrain to a LD cycle [7] . P. andruzzii possesses truncation mutations in two candidate circadian photoreceptors, tmt opsin and melanopsin , which are thought to contribute to its ‘blind’ circadian phenotype [7] . Our preliminary analysis of tmt opsin sequences reveals full-length coding regions in several cave populations, with amino-acid changes present outside of key opsin functional domains. This indicates that evolutionary changes in circadian clock function are likely to differ in each cave species, although elements of the circadian light input pathway are obvious ‘targets’ for evolutionary change. Could there be any selective advantage for cavefish of ‘perceiving’ sustained light exposure? Light has a profound impact on gene expression and physiology in fish [25] , [26] . Consequently, one would predict that isolation in a cave would influence a wide range of biological processes. Previous studies in teleosts have shown that transcriptional activation of DNA repair enzymes is light-dependent [23] , [25] , [26] , [40] . In Astyanax cave populations, two genes involved in DNA repair, CPD phr and ddb2 , show raised basal levels of expression, as with other light-regulated genes we have examined. In field samples from Chica Cave, this increase in CPD phr and ddb2 expression is more exaggerated with quite a dramatic increase, not only over surface fish, but also compared with cave strains within the lab. Presumably such a large change provides some selective advantage to those animals living under these conditions. At first, the result with CPD photolyase might seem rather counterintuitive. Proteins involved in photoreactivation, such as CPD photolyase, are directly light activated, as a key step in the DNA repair process. However, CPD photolyase is also known to bind to sites of DNA damage in the absence of light and subsequently, recruit additional DNA repair proteins, such as those involved in nucleotide excision repair, to the damaged site [44] , [45] . It is a reasonable hypothesis, therefore, that CPD photolyase in wild cave populations might have a functional role in DNA repair, even within the complete darkness of the cave. Quantification of DNA repair within animals kept in the lab revealed that cavefish are indeed more efficient than surface fish at repairing damaged DNA. It is therefore plausible to suggest that the greater expression of DNA repair genes in the wild cave populations would also lead to enhanced enzyme activity. The cave environment, and especially that of the trapped water, is particularly harsh. An animal that has ‘lost’ the ability to activate DNA repair events due to the lack of light or to other environmental factors, such as altered pH or oxygen levels of the water, might be at risk of significantly increased DNA damage, potentially resulting in an increase in deleterious mutational events. Interestingly, recent studies have shown that CPD photolyase can interact directly with the CLOCK protein to reduce CLOCK/BMAL-dependent transactivation and dramatically repress the mammalian circadian oscillator [46] . It is possible that the high levels of CPD photolyase we observe in the cave could have the same effect and be, in part, responsible for the highly repressed levels of clock function we observe in the wild. In general, the cave strain clock appears significantly less robust than that found in equivalent surface individuals. By tonically activating light-dependent signalling pathways and increasing DNA repair activity, individuals in the cave would reduce deleterious mutational events. This process would provide a clear advantage to those animals possessing this trait, even at the expense of possessing a damped or disrupted circadian pacemaker. Biological materials Adult surface fish, Pachón, and Chica cavefish, derived from fish from the laboratory of Dr William Jeffery at the University of Maryland, and adult surface x Pachón F1 hybrids, derived from crosses made in University College London, were maintained in the laboratory at 22–25 °C on a 14/10-hour photoperiod. All animals were maintained in a Home Office approved facility and handled in accordance with the Animal Welfare Act of 2006. Astyanax mexicanus cell lines were generated from 24-hour post-fertilization embryos obtained by temperature-induced spawning from surface fish, Pachón and Chica cavefish. These cell lines were cultured at 28 °C in L15 media containing 15% FCS, penicillin (100 U ml −1 ), streptomycin (100 μg ml −1 ) and gentamicin (50 μg ml −1 ), and used in this study for the construction of 5′ and 3′ RACE libraries described below. Cloning of Astyanax mexicanus clock genes To isolate clock genes from Astyanax mexicanus , PCR primers were designed to per1 , per2 , cry1a , tmt opsin , tef1 , CPD photolyase and ddb2 , by aligning sequences from several different teleost species ( Supplementary Table S1 ). PCR products of the appropriate size were obtained from Astyanax fin, embryo or cell line RNA by reverse transcriptase polymerase chain reaction (RT–PCR) and subcloned into pGEM-T Easy (Promega). These DNA fragments were sequenced using BigDye Terminator v1.1 (Applied Biosystems) and their identity determined by the BLAST algorithm. These sequences were then used to design primers for rapid amplification of cDNA ends (RACE) PCR to obtain full-length cDNAs. 5′ and 3′ RACE libraries were constructed using poly A + -purified RNA from Astyanax embryonic cell lines (described above) and the SMART RACE cDNA Amplification Kit (Clontech). 5′ and 3′ RACE PCR products were amplified with Advantage II Polymerase (Clontech), subcloned and sequenced as above. These RACE sequences, along with RT–PCR products, were assembled in CodonCode Aligner (CodonCode Corporation) and used to design primers ( Supplementary Table S1 ) to obtain full-length sequences for per1 and cry1a . Full-length coding regions were then amplified by RT–PCR from different Astyanax populations, and at least three independent clones for each gene were sequenced. Astyanax nucleotide sequences have been deposited into Genbank. Alignments of predicted amino-acid sequences from surface and cavefish populations were created using the ClustalW algorithm in MegAlign (DNASTAR). Quantitative PCR For time series experiments in the laboratory, adult fish maintained at 22–25 °C were exposed to a 12/12-hour LD cycle for 7 days before transfer into constant darkness. Caudal fin clips were taken at 6-hour intervals, with each fin placed in a separate tube of TRIzol Reagent (Invitrogen), homogenized and stored at −20 °C. Total RNA was extracted following the manufacturer’s instructions. For acute light pulse experiments, adult fish were maintained on a LD cycle as above, but given a 3-hour light pulse at ZT16 on day 7, or kept in the dark as a control. Fin samples were then collected, homogenized and total RNA extracted as above. cDNA was synthesized from 2 μg of RNA using Superscript II Reverse Transcriptase (Invitrogen) with random hexamers and oligo dT primers. Each fin sample was analysed in triplicate by qPCR using SYBR Green JumpStart Taq ReadyMix (Sigma) and gene-specific primers ( Supplementary Table S1 ) at a concentration of 500 nM. Δ C t was determined using rpl13 α as a reference gene, and as C t values for rpl13 α were remarkably consistent between all Astyanax populations, relative expression levels between surface fish and cavefish were compared directly using the ΔΔ C t method. Behavioural studies Single adult surface fish, Pachón, and Chica cavefish were maintained in the laboratory at 22±1 °C and entrained to a 12/12-hour photoperiod for at least 7 days in separate tanks measuring 41 × 20 × 25 cm. Near infrared cameras (Sony CCTV CCD 420 TVL) with a 3.6 mm wide-angle lens were mounted in front of each tank to allow the recording of the fish in light and dark conditions. Analogue video signal was recorded and compressed with Xvid MPEG4 codec through a Steren USB external S-video card using Debut Video Capture software (NCH software) at 30 frames per second, with a resolution of 640 × 480 pixels. Fish were recorded for 2 days in LD before transfer into constant darkness and recorded for a further 2 days. Videos were analysed with the movement quantification module of videotrack software (ViewPoint), with a detection threshold of 15 and a threshold of analysis (‘burst’) of 500. For each fish, the time spent swimming faster than 5 cm s −1 in a 30-min bin was taken. Activity, binned over 30 min, was normalized to the mean activity level for each fish, and the mean of four or more normalized activity levels were plotted. Data was analysed for rhythmicity by autocorrelation (with 95% confidence), and estimates of period were determined by spectral resampling in MATLAB (Mathworks) [38] . ELISA For quantification of DNA repair activity, caudal fin clips were taken from adult fish (which had been maintained on a 14/10-hour LD cycle at 22–25 °C) at ZT23.5. The fins were washed once in PBS-containing penicillin (200 U ml −1 ) and streptomycin (200 μg ml −1 ), and either exposed to UV light of 1 mJ cm −2 or kept in the dark as an undamaged control. Fins were subsequently incubated in L15 media containing 15% FCS, penicillin (100 U ml −1 ), streptomycin (100 μg ml −1 ) and gentamicin (50 μg ml −1 ). At 0.5 and 24 h after the UV pulse, fins were immediately frozen at −80 °C. Genomic DNA was extracted using the GeneJet Genomic DNA kit (Fermentas). Cyclobutane pyrimidine dimer photoproducts (CPDpp) were detected by ELISA using TDM-2 monoclonal antibodies (Cosmo Bio) following a modified protocol [41] . Denatured genomic DNA (diluted to 0.2 μg ml −1 in PBS, 10 ng per well) was bound in quadruplicate to 96-well polyvinylchloride flat-bottom plates, pre-coated with 0.003% protamine sulphate, overnight at 37 °C. Plates were washed PBS-Tween (0.05%) before addition of TDM-2 diluted in PBS (1:1,000) to each well and incubated for 30 min at 37 °C. Control wells containing DNA were incubated in PBS in the absence of TDM-2 antibodies. After washing with PBS-Tween (0.05%), the bound antibody was detected by incubation with biotinylated F(ab’)2 fragment of goat anti-mouse IgG (1:2,000; Zymed, Life Technologies) for 30 min with 37 °C, washed with PBS-Tween (0.05%) and then incubated with peroxidase–streptavidin (1:10,000; Zymed, Life Technologies) for a further 30 min at 37 °C. The plate was incubated with o-Phenylenediamine for 30 min at 37 °C to detect peroxidase activity; after stopping the reaction with H 2 SO 4 , absorbance was measured at 492 nm. Data are presented as a percentage of CPD photoproducts remaining, as calculated by the ratio of the respective OD after 24 h and 0.5 h after UV light pulse. Field studies In the Micos River, adult fish were captured using baited fish traps and nets, 2–3 days prior to the sampling period. The fish were then placed in large, perforated tubs, open to natural water flow and allowed to float within the main stream of the river. An individual tub was set up for each time point to reduce any possible disturbance to other animals during the experiment. Nighttime samples were collected using head torches with dim red light. Caudal fin clips were taken at six time points per day over 2 days, with each fin placed in a separate tube of TRIzol Reagent (Invitrogen), homogenized, immediately placed on ice and later stored at −20 °C. Total RNA was extracted from individual samples, cDNA synthesized and qPCR carried out as described above. Cave samples were collected using a similar approach, with individual open tubs being floated within the cave ponds. Animals were collected (typically 40 fish or more) using dim red light, and sampling was performed in a location away from the main body of fish to reduce any possible disturbance. All clipped animals were kept in a separate container away from the experimental individuals and were not released back into the main body of water until the end of the study. Water quality was monitored using a Multi-Parameter TROLL 9,500 probe (In-Suit.) suspended in the water column next to the collected fish. This device provided continuous measurements of water temperature, barometric pressure, pH, dissolved oxygen and nitrates. Statistical analysis The data in this study are presented as the mean±s.e.m. ( n >3) and were analysed using a Student’s t- test or analysis of variance ( http://www.physics.csbsju.edu/stats ), followed by Newman–Keuls multiple comparison posttest in GraphPad Prism (GraphPad Software). P <0.05 was considered significant. Accession codes: Sequences have been deposited on GenBank nucleotide database under accession numbers: KF737843 – KF737860 . How to cite this article: Beale, A. et al. Circadian rhythms in Mexican blind cavefish Astyanax mexicanus in the lab and in the field. Nat. Commun. 4:2769 doi: 10.1038/ncomms3769 (2013).